Reply To: Comments on identifying causal relationships in nonlinear dynamical systems via empirical mode decomposition 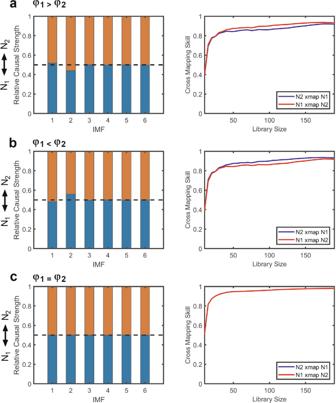Fig. 1: Causal patterns of adult-recruitment model in various settings of environmental forcing. The adult-recruitment model is a 5-variate differential equation to simulate the Moran effect that the populations of two independent species N1and N2are driven by the external forcing of the environmental noise. With appropriate mathematical deductions (see supplementary information), we found that N1and N2are causally coupled with each other and the causal strengths between them are driven by the ratio of environmental forcing. For simplicity, the parameters were given here asr1= 3.4,s1= 0.4, andD1= 3, as well asr2= 3.4,s2= 0.4, andD2= 3. The initial value ofRandNwas set as 1 and 0.5, respectively in both pairs. The model was simulated for 10,000 iterations and the last 200 data points of N1and N2were extracted for causal analysis with causal decomposition and convergent cross mapping (CCM) method. The parameters for causal decomposition and CCM method were the same with Chang et al1. (i.e., noise level = 0.085, ensemble number = 1000, and embedding dimension for CCM = 4). We tested the causal decomposition and CCM results in the various settings of environmental forcing at (a),φ1= 0.6 andφ2= 0.5; (b),φ1= 0.5 andφ2= 0.6; and (c),φ1= 0.5 andφ2= 0.5. As expected, the causal decomposition showed a correct direction of coupling in these different settings of environmental forcing. CCM also showed a consistent pattern of bi-directional coupling between N1and N2in three settings (statistical tests of Kendall’s τ test and Fisher’s Δρ Z score for the significance of convergence of cross mapping showedp< 0.05 in all settings.). Further information on research design is available in the Nature Research Reporting Summary linked to this article.